Dynamics of a producer-freeloader ecosystem on the brink of collapse Ecosystems can undergo sudden shifts to undesirable states, but recent studies with simple single-species ecosystems have demonstrated that advance warning can be provided by the slowing down of population dynamics near a tipping point. However, it is unclear how this ‘critical slowing down’ will manifest in ecosystems with strong interactions between their components. Here we probe the dynamics of an experimental producer-freeloader ecosystem as it approaches a catastrophic collapse. Surprisingly, the producer population grows in size as the environment deteriorates, highlighting that population size can be a misleading measure of ecosystem stability. By analysing the oscillatory producer-freeloader dynamics for over 100 generations in multiple environmental conditions, we find that the collective ecosystem dynamics slow down as the tipping point is approached. Analysis of the coupled dynamics of interacting populations may therefore be necessary to provide advance warning of collapse in complex communities. Climate change and overexploitation of natural resources are altering many of the earth’s ecosystems, often leading to habitat loss and species extinction. These regime shifts in ecological systems can occur without obvious warning; and once they have transpired, they may be extremely difficult to reverse, even after the agent that caused them is identified and removed [1] , [2] , [3] , [4] , [5] , [6] . This irreversibility is a consequence of the ecosystem undergoing a critical transition, in which it switches from one stable state to another. Once this happens, the feedback loops that stabilize the new state make it difficult to reverse the transition, leading to memory effects or hysteresis [1] , [2] , [7] . As ecosystems approach such critical transitions they may often lose resilience, making it easier for external perturbations to induce a regime shift [8] . Given the negative consequences of these unwanted regime shifts, there is a desire to measure the stability of ecosystems and identify early warning indicators preceding catastrophic transitions. Recently, there has been growing interest in using bifurcation theory [7] , [9] , [10] , [11] and the signatures of critical slowing down [12] , [13] (a phenomenon well studied in physics [14] , [15] and many other fields [16] , [17] , [18] , [19] , [20] , [21] , [22] ) as a paradigm to understand the dynamics before transitions between alternative stable states in ecosystems. Theory further suggests that the loss of resilience of an ecosystem as it approaches a tipping point should be accompanied by a slowing down of the collective dynamics of the ecosystem [1] , [8] , [23] , [24] , [25] . This prediction has been confirmed in single-species laboratory microcosms, where critical slowing down and its indirect signatures (for example, increases in population variability and the correlation of fluctuations) have been observed [26] , [27] , [28] . In parallel with the studies of simple laboratory populations, early warning indicators based on critical slowing down have been studied in models of complex ecosystems [2] , [6] , [26] , [29] , [30] . Indeed, it is expected that sudden transitions will be common in ecological networks with multiple interacting species [2] . Theoretical analysis of concrete ecosystems with either two [23] or three [29] strongly interacting species concluded that the collapse of more complex ecosystems may also be preceded by critical slowing down—in this case manifested as the dominant eigenvalue of the community matrix approaching zero [30] (or one, for temporally discretized dynamics [31] ). Encouragingly, recent experiments of exceedingly complex lake ecosystems indicate that the effects of critical slowing down may be seen by investigating the dynamics of individual species, or indirect reporters of the presence of other species [32] , [33] . Nevertheless, how critical transitions take place in complex ecological networks is still poorly understood; for instance, as to how the inter-specific interactions within the ecosystem [34] affect the collective dynamics on the brink of a regime shift, or which particular indicator will exhibit the strongest signatures of critical slowing down. To address these questions, and to understand how early warning indicators behave in ecosystems with strong interactions between species, we set out to study the dynamics of a laboratory producer-freeloader ecosystem consisting of two yeast strains with different phenotypes. Our producer-freeloader ecosystem consists of two different strains of budding yeast ( Saccharomyces cerevisiae ) growing on sucrose. Budding yeast requires the enzyme invertase to break down sucrose into glucose and fructose. Invertase is secreted into the periplasmic space between the cell membrane and the cell wall. Due to this secretion outside of the cell, 99% of the glucose and fructose diffuse away from the cell that produced them, and can be consumed by other cells in the population [35] . In our experiments, the ‘producer’ strain expresses the SUC2 gene that encodes for invertase production; the second yeast strain, the ‘freeloader’ lacks this gene and does not contribute to the breakdown of sucrose. Thus, the freeloader population exploits the producer population by consuming glucose and fructose without paying the metabolic cost associated with their production. This experimental system has been previously characterized as a model of the public-goods evolutionary game dynamics between cooperators and cheaters [35] , [36] , [37] , [38] , [39] . This evolutionary intra-species interaction is a particular realization of a more general ecological interaction where one species (a producer) produces a resource that is also consumed by individuals that benefit from it but which have not contributed to its production (freeloaders). Mathematically, the cooperator–cheater dynamics has been shown to be equivalent to the dynamics between producers and freeloaders (or prey and predators) [36] , [40] . Collapse of an experimental producer-freeloader ecosystem Based on prior experiments with monocultures of the producer strain in sucrose media [27] , we expected our producer-freeloader ecosystem to exhibit a critical collapse as the environment deteriorates. To test this, we grew replicate co-cultures of the two yeast strains in sucrose media, and subjected the cultures to multiple daily cycles of growth-dilution (see Methods). This experimental design naturally introduces an experimentally tunable dilution factor (DF), akin to a mortality rate, which was our control parameter for environmental deterioration [27] , [36] . We followed the ecosystems for nine days and measured the density of the producer and freeloader populations after each growth-dilution cycle. Our observations are consistent with the presence of a tipping point in our ecosystem located around a DF of 2,000: below that DF the populations found a stable equilibrium, but when the DF was increased beyond this value, the populations collapsed and went extinct ( Fig. 1 ). 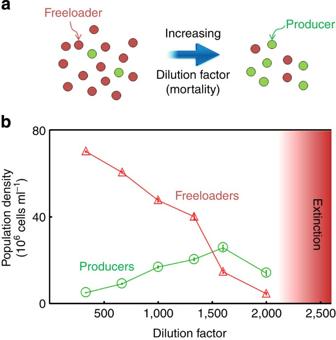Figure 1: Environmental deterioration leads to a surprising increase in the producer population size preceding collapse of a producer-freeloader ecosystem. (a) Yeast populations were grown in sucrose media and subjected to a range of daily dilution factors. Experiments were started with identical initial concentrations of producers (which carry the gene SUC2 required for sucrose break down) and freeloaders (SUC2 knockouts). (b) The equilibrium population density of the producer (green) and freeloader (red) populations as a function of dilution factor. Error bars represent s.e.m. (n=20). The producer population size increases as the environment deteriorates, highlighting that population size is not always a reliable indicator of population health. Figure 1: Environmental deterioration leads to a surprising increase in the producer population size preceding collapse of a producer-freeloader ecosystem. ( a ) Yeast populations were grown in sucrose media and subjected to a range of daily dilution factors. Experiments were started with identical initial concentrations of producers (which carry the gene SUC2 required for sucrose break down) and freeloaders (SUC2 knockouts). ( b ) The equilibrium population density of the producer (green) and freeloader (red) populations as a function of dilution factor. Error bars represent s.e.m. ( n =20). The producer population size increases as the environment deteriorates, highlighting that population size is not always a reliable indicator of population health. Full size image In previous experimental studies in monocultures [26] , [27] , [28] , the population size always declined with environment deterioration. In particular, this was the case for cultures of our producer strain in isolation [27] . In contrast, here we found that in the face of competition with the freeloader strain (whose population size does show the expected decline) the producer population increased in size as the environment deteriorated, and was maximal in the proximity of the tipping point ( Fig. 1b ). This increase in population size of the producer population as the environment deteriorates is a consequence of the nonlinear coupled dynamics in the system ( Supplementary Fig. 1 ); at high DFs, the lower density of freeloaders leads to weaker competitive interactions and allows for less hindered growth of the producers. Species interactions may therefore lead to counter-intuitive changes at the ecosystem level as the environment deteriorates. Thus, in contrast to simple single-species ecosystems, changes in the population size of any individual species are not necessarily a reliable indicator of loss of resilience in a complex ecosystem. Loss of ecological resilience may be foreseen by critical slowing down As a warning indicator of tipping points in an ecosystem, critical slowing down is manifested in the collective dynamics of the whole ecosystem; in particular, it is characterized by the dominant eigenvalue of the linearized discrete dynamics around equilibrium (that is, the interaction matrix [31] ). The absolute value of the dominant eigenvalue of the interaction matrix describing the discrete dynamics is expected to approach |λ dom |=1 as the system approaches a critical transition [23] . To observe the coupled dynamics in our population, we plotted the trajectories followed by the ecosystem on the producer-freeloader phase plane ( Fig. 2 ). Consistent with previous experiments [36] , the trajectories spiralled to an equilibrium at which the two populations coexist. The observed damped oscillations is a hallmark of the coupled dynamics resulting from the interactions between producers and freeloaders [41] , [42] , [43] , [44] , [45] , [46] , [47] . Given our experimental resolution and the level of noise, we cannot entirely rule out the possible existence of a very small limit cycle, but our data of population trajectories at equilibrium in a longer experiment ( Supplementary Fig. 2e ) as well as the dynamics in simulations ( Supplementary Fig. 3 ) indicate that our system converged to a stable fixed point. We estimated the equilibrium point in the producer-freeloader phase plane ( Supplementary Fig. 4 ), and fit the spirals to a first-order multivariate autoregressive model to obtain an estimate for the interaction matrix, from which the eigenvalues could be calculated (see Methods). As expected from the spiralling trajectories, the eigenvalues had both a real and an imaginary component. For the trajectory plotted in Fig. 2 , corresponding to a DF of 1,333, we found λ 1,2 = |λ|e ± iθ , where |λ| =0.83±0.11 and θ =39°±6°. For these spiralling trajectories, the magnitude of the eigenvalue |λ| specifies how rapidly the trajectories radially converge to the equilibrium, whereas the angle θ reflects how quickly the trajectories spiral tangentially around the equilibrium. The theory of critical slowing down predicts that |λ| should increase, approaching ~1 as the ecosystem approaches the tipping point of a critical transition. This means that as the environment deteriorates it takes longer for the two subpopulations to reach equilibrium [23] . 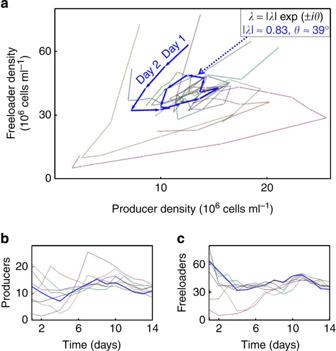Figure 2: The coupled spiral dynamics of the producer-freeloader ecosystem can be characterized by complex eigenvalues. (a) The dynamics of the population density can be visualized as trajectories in the producer-freeloader phase plane. Replicate populations were grown from 30 different starting densities with a daily dilution of 1,333 for 14 days. Selected trajectories are coloured consistently on the three plots, with remaining trajectories shown in light grey. The indicated blue trajectory has complex eigenvaluesλ=0.83e±i39°. The individual dynamics of the producers (b) and the freeloaders (c) are plotted as a function of time (both are expressed in units of 106cells ml−1). Figure 2: The coupled spiral dynamics of the producer-freeloader ecosystem can be characterized by complex eigenvalues. ( a ) The dynamics of the population density can be visualized as trajectories in the producer-freeloader phase plane. Replicate populations were grown from 30 different starting densities with a daily dilution of 1,333 for 14 days. Selected trajectories are coloured consistently on the three plots, with remaining trajectories shown in light grey. The indicated blue trajectory has complex eigenvalues λ =0.83 e ± i 39° . The individual dynamics of the producers ( b ) and the freeloaders ( c ) are plotted as a function of time (both are expressed in units of 10 6 cells ml −1 ). Full size image To test these theoretical predictions, we subjected our producer-freeloader ecosystems to eight different DFs, ranging from 50 to 1,600. Thirty replicate ecosystems were tracked for each DF. As expected, the absolute magnitude of the eigenvalue increased substantially as the environmental quality decreased, and approached |λ| =1 just before population collapse ( Fig. 3 ). Thus, our direct observation of critical slowing down in an experimental producer-freeloader ecosystem lends support to the linearization approach in assessing community stability and species interactions [31] , as well as using the dominant eigenvalue of the interaction matrix as a warning signal in multi-species ecosystems. We are not aware of any theoretical predictions regarding the behaviour of θ (argument of eigenvalues) as the tipping point is approached, and indeed we did not observe any noticeable change in θ ( Supplementary Fig. 2e ). 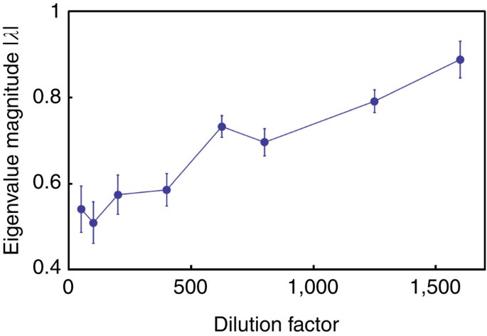Figure 3: Consistent with critical slowing down, the magnitude of the complex eigenvalues increases as ecosystem collapse is approached. Thirty replicate populations with varying initial conditions were grown at each of eight different daily dilution factors. Their spiralling trajectories were analysed to estimate their eigenvalues (generally a pair of complex conjugates). As predicted by theory, the magnitude of the eigenvalues increases and approaches one as the environment deteriorates. Dilution factors above 1,600 were not assessed due to the difficulty of calculating eigenvalues from very noisy data (see DF 2,000 inFig. 4). Error bars represent standard error and were obtained by bootstrapping the experimental trajectories as well as the location of the fixed point with 50 resamplings. Figure 3: Consistent with critical slowing down, the magnitude of the complex eigenvalues increases as ecosystem collapse is approached. Thirty replicate populations with varying initial conditions were grown at each of eight different daily dilution factors. Their spiralling trajectories were analysed to estimate their eigenvalues (generally a pair of complex conjugates). As predicted by theory, the magnitude of the eigenvalues increases and approaches one as the environment deteriorates. Dilution factors above 1,600 were not assessed due to the difficulty of calculating eigenvalues from very noisy data (see DF 2,000 in Fig. 4 ). Error bars represent standard error and were obtained by bootstrapping the experimental trajectories as well as the location of the fixed point with 50 resamplings. Full size image Indirect early warning indicators at the single-species level Previous analyses of natural ecosystems had indicated that individual species may exhibit behaviours consistent with critical slowing down as the ecosystem approaches a bifurcation [32] . Mathematical analysis of the dynamics of a general two-species ecosystem reveals that the variability in the fluctuations of population density of each species is expected to diverge when |λ| approaches 1 near a tipping point [31] ( Supplementary Note 1 ). Therefore, statistical indicators based on the size of fluctuations in the population density of individual species may provide indirect signatures of critical slowing down at the ecosystem level. To test this, we measured the coefficient of variation (CV) between replicates on the final day of the experiment for both the producer and freeloader populations (see Methods). We found that the CV increased sharply with rising DFs for both producer and freeloader populations ( Fig. 4 ). Therefore, variability in the density of either species across replicates provides an early warning signal of the approaching tipping point in our producer-freeloader ecosystem, even when the equilibrium population density increases (which is the case for our producer population). 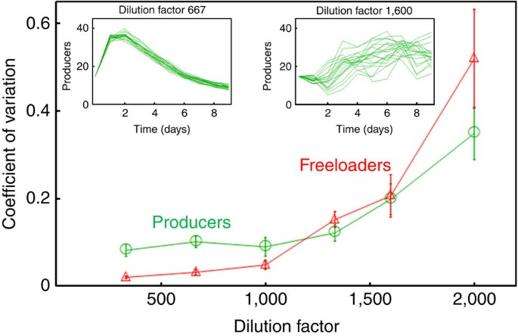Figure 4: Coefficient of variation of both subpopulations increases as the environment deteriorates due to increasing dilution factor. The coefficient of variation (CV) measured for both producer (green) and freeloader (red) populations as a function of dilution factor. Populations were grown from the same initial density of producers and freeloaders, and the coefficient of variation across the 20 replicates for each dilution factor was measured on the final day of the experiment (day 9). Inset figures represent the time series of the producer density (measured in 106cells ml−1) of each replicate at a low dilution factor (left panel) and a high dilution factor (right panel). Similar results were found for the freeloader populations. Error bars are standard errors obtained by bootstrapping with 100 resamplings. Figure 4: Coefficient of variation of both subpopulations increases as the environment deteriorates due to increasing dilution factor. The coefficient of variation (CV) measured for both producer (green) and freeloader (red) populations as a function of dilution factor. Populations were grown from the same initial density of producers and freeloaders, and the coefficient of variation across the 20 replicates for each dilution factor was measured on the final day of the experiment (day 9). Inset figures represent the time series of the producer density (measured in 10 6 cells ml −1 ) of each replicate at a low dilution factor (left panel) and a high dilution factor (right panel). Similar results were found for the freeloader populations. Error bars are standard errors obtained by bootstrapping with 100 resamplings. Full size image Several other indicators of critical slowing down have been proposed theoretically and some observed experimentally in monocultures [1] , [2] , [26] , [27] , [28] . They include the deterministic return time following a pulse perturbation and the lag-1 autocorrelation of the fluctuations of the population density. In our experiments with a relatively small sample size, both the deterministic return time and the lag-1 autocorrelation based on single-species time series failed to produce statistically significant increases with an increasing DF ( Supplementary Figs 2c,d and 5 ). In a previous experiment with monocultures of the producer population [27] , we observed a clear increase in the CV, lag-1 autocorrelation and return time before population collapse. Our experiments and mathematical analysis reported here suggest that certain warning indicators based on a single species may fail in the presence of interactions between species ( Supplementary Notes 1 and 2 ). This failure of some indicators based on single-species data highlights the importance of understanding species interactions in the application of early warning indicators to complex ecosystems; it also supports the notion that stability is a property of the entire community instead of its constituent species [48] . Although properties of the whole community may not always be inferred from a single species, replicate laboratory ecosystems can help to elucidate the warning indicators that will be most useful and reliable in real-world settings. Our study represents an initial characterization of population dynamics near a regime shift in an ecological network with strong inter-species interactions. Due to the impracticality of assessing unstable systems, it is difficult to determine the exact nature of the transition. Our model predicts a Hopf bifurcation ( Supplementary Fig. 3 ), which exhibits critical slowing down near its tipping point [6] . Although our system is two-dimensional, it is worth noting that bifurcations in higher dimensions can be extraordinarily rich and complex [9] . Even in low-dimensional systems, not all bifurcations lead to critical slowing down, and regime shifts may occur with no warning [49] , [50] , [51] . On the other hand, recent theoretical studies have pointed out that, in some instances, critical slowing down can be detected even in the absence of any critical transitions [50] , [52] , [53] . In spite of these potential caveats in using critical slowing down to forecast ecological regime shifts, our experiments demonstrate that it may be possible to observe the dominant eigenvalue of the interaction matrix increasing and approaching 1 before the collapse of a producer-freeloader ecosystem, and provide support to the utility of critical slowing down as a warning signal in multi-species ecosystems [23] , [48] , [54] . We also recognize that there are other alternative indices based on the interaction matrix, which may prove useful in quantifying the transient dynamics [48] , [55] . In many ecosystems it may not be possible to study the collective dynamics of the whole system and obtain the eigenvalues, as that would require tracking the dynamics for each of the interacting species. However, our optimism in understanding complex ecosystems come from the belief that many ecosystems may consist of loosely coupled units with low dimensionality [56] . Recent experiments in a whole-lake ecosystem [32] provided evidence that some warning indicators can be observed based on time series of individual species within a multi-species ecosystem. In spite of this favourable empirical example, we caution that analysing any single species in an ecosystem does not necessarily provide reliable warning indicators, especially when the coupling between species leads to oscillatory dynamics, as seen in this study. Our study underscores the necessity of characterizing species interactions and collective dynamics when applying early warning signals to complex ecosystems. More quantitative studies in multi-species systems, especially in spatially extended contexts [24] , [57] , [58] , [59] , will shed light on how to monitor a complex ecosystem to maximize the utility of early warning indicators. Strains The producer strain, JG300A [35] , is derived from BY4741 strain of S. cerevisiae (mating type a, EUROSCARF) that has a wild-type SUC2 gene. It constitutively expresses YFP from the ADH1 promoter (inserted using plasmid pRS401, with a MET17 marker), and also has a mutated HIS3 ( his3Δ1 ). The freeloader strain, JG210C [35] , is a SUC2 deletion strain (EUROSCARF Y02321, SUC2::kanMX4 ) of S. cerevisiae . It constitutively expresses dTomato from the PGK1 promoter (inserted using plasmid pRS301, with a HIS3 marker). Culture growth The growth medium was composed of synthetic media (YNB and CSM-his; Sunrise Science, California), 2% sucrose, 0.001% glucose and 8 μg ml −1 histidine [36] . Cells were cultured in 200 μl of media within the 60 internal wells of a Falcon flat-bottom 96-well plate (BD Biosciences, California), with the 36 external wells filled with 200 μl growth media [36] . The plates were incubated at 30 °C, while being shaken at 800 r.p.m. During incubation, the plates were covered with Parafilm as well as the plate cover. Cultures were subject to growth-dilution cycles [36] , where cells were allowed to grow for 23.5 h and then diluted by a predetermined DF. The cultures were then incubated again, beginning a new day’s cycle. Measurement of population densities The optical density of each culture at 620 nm was measured with a Thermo Scientific Multiskan FC microplate spectrophotometer, following the end of each growth period [27] . To measure the fractions of each population, at the end of each growth period a portion of cells from each well (typically 5 μl, unless the low density conditions made it necessary to transfer larger volumes) was transferred to a new plate containing 200 μl sterile Cellgro PBS buffer (Mediatech, Virginia). These samples were then analysed at a BD LSRII-HTS flow cytometer operating in high throughput mode, where we determined the ratio between the producer and freeloader strains, distinguished by their fluorescence emissions [36] . Given the total density and the strain ratio, the densities of the producer and freeloader populations were readily calculated. Calculation of CV CV was calculated for each subpopulation by dividing the standard deviation of the final-day population by the final-day sample mean. Populations that were dying or dead were filtered out, as per Supplementary Note 3 . Errors were estimated by bootstrapping, with 100 resamplings. Calculation of eigenvalues The eigenvalues of the system are calculated by linearizing the dynamics of the trajectories around the equilibrium point. Because we observe the producer and freeloader populations in discrete time intervals (once per day), we can model their motion on the producer-freeloader phase plane by a difference equation: where ( x t , y t ) is the vector containing the producer ( X ) and freeloader ( Y ) populations on day t . ( X*, Y* ) is the equilibrium point of the trajectory, and J is the 2 × 2 Jacobian matrix (or ‘interaction matrix’) that describes the dynamics on the producer-freeloader phase plane. Each day, this Jacobian matrix is applied to the previous day’s population vector ( X t , Y t ) to generate the next day’s set of producer and freeloader densities ( X t +1 , Y t +1 ). Notice that this is a linear transformation, which is not an exact reflection of the nonlinear dynamics for the entire phase plane. However, in the vicinity of a fixed point (as in our experiments), we may choose to retain only the first-order terms of the Taylor expansion of the true transformation. The ensuing linear system is thus a reasonable approximation to our spiralling trajectories near the fixed point. Once we determine our best estimate for the matrix J , we can perform an eigendecomposition to calculate its eigenvalues (assuming that the Jacobian matrix is not defective): where λ 1 and λ 2 are the eigenvalues of J , and P is the matrix whose columns are the two eigenvectors of J . To determine J from our experimental data, we took two approaches in fitting the trajectories as per equation (1), which are further described in Supplementary Note 4 . How to cite this article: Chen, A. et al. Dynamics of a producer-freeloader ecosystem on the brink of collapse. Nat. Commun. 5:3713 doi: 10.1038/ncomms4713 (2014).